Flexible and transparent all-graphene circuits for quaternary digital modulations In modern communication systems, modulation is a key function that embeds the baseband signal (information) into a carrier wave so that it can be successfully broadcasted through a medium such as air or cables. Here we report a flexible all-graphene modulator circuit with the capability of encoding a carrier signal with quaternary digital information. By exploiting the ambipolarity and the nonlinearity in a graphene transistor, we demonstrate two types of quaternary modulation schemes: quaternary amplitude-shift keying and quadrature phase-shift keying. Remarkably, both modulation schemes can be realized with just 1 and 2 all-graphene transistors, respectively, representing a drastic reduction in circuit complexity when compared with conventional modulators. In addition, the circuit is not only flexible but also highly transparent (~95% transmittance) owing to its all-graphene design with every component (channel, interconnects, load resistor and source/drain/gate electrodes) fabricated from graphene films. Physically compliant electronics with the capability to conform to a non-planar surface is a field of rapidly growing interest due to the numerous possibilities it offers. Applications ranging from flexible solar cells [1] , displays [2] , e-papers [3] , wearable electronics [4] and biomedical skin-like devices [5] , [6] open up new opportunities in the field of electronics. However, nearly all flexible electronic devices require an external power supply and data communication modules, and the lack of portability can severely limit the functionality of various applications. To drive the field forward, three key challenges need to be addressed: a means to generate or store power (for example, flexible batteries or power generators), a data collecting scheme (for example, flexible sensors) and a system to transmit and receive the collected data (for example, flexible wireless communication scheme). Recent advances in the field have led to notable progress in the two areas of flexible power [7] , [8] and flexible sensors [5] , [6] . However, designing and manufacturing a flexible wireless communication system is still a challenge owing to material constraints. Conventional organic polymers [9] , amorphous silicon [10] , or oxide-based thin film transistors [11] , [12] show only modest performance in this area owing to their limited carrier mobilities. In this regard, graphene is the ideal material for flexible high-speed communication systems owing to its unique electronic and physical properties, including high carrier mobility [13] , ambipolarity [14] , [15] , transparency [16] and mechanical flexibility [17] . For example, graphene transistors have achieved unity gain cutoff frequencies of up to 300 GHz (refs 18 , 19 ). Graphene was also used as the channel and the gate material for flexible transistors owing to its mechanical flexibility [20] , [21] . Despite graphene transistors' low on/off ratio that limits their usage in the digital/logic applications, they are attractive in the analogue/radio frequency applications due to graphene's extremely thin structure that allows shorter scaling of channel length without the adverse short channel effects [22] . Beyond individual transistor, pioneering works on graphene analogue electronics led to the demonstration of graphene-based frequency doublers [23] , [24] , [25] , mixers [26] , [27] and modulators [24] , [28] , [29] on rigid substrates. Graphene mixers were shown to effectively suppress odd-order intermodulations by exploiting the symmetric character of graphene transistors [26] . A high-performance mixer fabricated by integration of graphene transistors and passive components on a single silicon carbide wafer was also demonstrated [27] . Taking it one step further, several groups demonstrated binary digital modulation schemes (binary phase-shift keying (BPSK) and binary frequency-shift keying (BFSK)) with graphene transistors on rigid substrates [24] , [28] , [29] . Despite the remarkable progress, all previous graphene analogue circuits were demonstrated on rigid silicon substrates. A flexible digital modulation scheme, which is the key building block for flexible high-speed data communication, has not been realized using graphene circuits. In addition, previous graphene binary modulators can only encode single bit of data per symbol. To this end, we demonstrate, for the first time, flexible and transparent all-graphene circuits for quaternary digital modulations that can encode two bits of information per symbol. The circuits are both flexible and transparent with every part of the circuit—including the transistor channels, the interconnects between transistors, the load resistance, and the source/drain/gate electrodes—fabricated with graphene only. The monolithic structure allows unprecedented mechanical flexibility and near-complete transparency that is not possible with either silicon or metal. This structure is possible because of graphene's unique property of being a zero-bandgap material retaining the property of both metal and semiconductor. Importantly, the ambipolarity of graphene transistors drastically reduces the circuit complexity when compared with silicon-based modulators. No more than a couple of transistors are required for the two quaternary modulation schemes demonstrated, whereas a multitude of transistors are required for conventional modulator circuits [30] , [31] . Modulation mechanism and transistor characteristics The basic modulation techniques map the information by varying up to three different parameters (amplitude, frequency and phase) of the carrier wave to represent the data. The most fundamental binary digital modulation techniques that correspond to each of these three parameters are binary amplitude-shift keying (BASK), BFSK, BPSK. Furthermore, by combining two or more binary modulation schemes, it is possible to extend this technique into quaternary digital modulation schemes such as quaternary amplitude-shift keying (4-ASK) and quadrature phase-shift keying (QPSK) [32] . Specifically, QPSK explores all four quadrants of the constellation, and it is the key building unit for highly efficient modulation techniques that are widely used in today's telecommunication standards such as Code division multiple access and Long-term evolution. The above-mentioned binary and quaternary digital modulation schemes are plotted in a polar constellation with the radial coordinate as the amplitude and the angular coordinate as the phase ( Fig. 1a ). Importantly, all of them can be realized by using all-graphene circuits on the flexible and transparent platform. 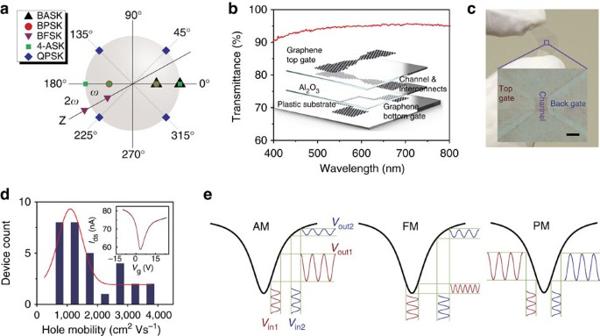Figure 1: Modulation mechanism and device characteristics of flexible and transparent all-graphene transistors. (a) A constellation diagram depicting five different digital modulation techniques demonstrated in this work. Thezaxis, representing the frequency, is included to show the frequency-modulated signals. (b) A plot of the transmittance as a function of the wavelength and an illustration of the all-graphene transistor structure (inset). (c) A photograph of graphene circuit on a transparent and bendable plastic substrate, and a microscopic image of an all-graphene transistor (inset). Scale- bar, 10 μm. (d) A histogram of the hole mobility extracted from 30 transistors and its Gaussian fit (red line). The inset is a plot of the ambipolar current as a function of gate voltage for a typical all-graphene transistor. Voltage across the drain and the source is 10 mV. (e) Illustrations of amplitude, frequency and phase modulation of a sinusoidal wave achieved by operating a single ambipolar graphene transistor at different gate biases. Figure 1: Modulation mechanism and device characteristics of flexible and transparent all-graphene transistors. ( a ) A constellation diagram depicting five different digital modulation techniques demonstrated in this work. The z axis, representing the frequency, is included to show the frequency-modulated signals. ( b ) A plot of the transmittance as a function of the wavelength and an illustration of the all-graphene transistor structure (inset). ( c ) A photograph of graphene circuit on a transparent and bendable plastic substrate, and a microscopic image of an all-graphene transistor (inset). Scale- bar, 10 μm. ( d ) A histogram of the hole mobility extracted from 30 transistors and its Gaussian fit (red line). The inset is a plot of the ambipolar current as a function of gate voltage for a typical all-graphene transistor. Voltage across the drain and the source is 10 mV. ( e ) Illustrations of amplitude, frequency and phase modulation of a sinusoidal wave achieved by operating a single ambipolar graphene transistor at different gate biases. Full size image Figure 1b (inset) shows the schematic of the all-graphene device fabricated on a bendable plastic (polyethylene naphthalate) substrate. The top, middle and bottom graphene layers form the top gate layer, the channel/interconnect layer, and the bottom gate layer, respectively. Two dielectric layers are deposited using an atomic layer deposition method to isolate the three graphene layers. The final device is highly transparent as shown in Fig. 1b (~95% transmittance; see Methods), and fully bendable as shown in Fig, 1c . The overall transmittance is higher than the expected value of 93% for tri-layer graphene [16] because the majority of the area is covered with only one layer of graphene. Under the optical microscope, the graphene devices can be identified by the contrast difference among the top gate, channel and bottom gate region of the all-graphene transistor ( Fig. 1c inset). The gate response curve was measured for each all-graphene transistors, and the yield was over 98%, with 64 out of 65 transistors being fully functional. Figure 1d (inset) shows a typical gate response curve from the fabricated all-graphene transistors. Slight shift in the charge neutrality point is observed owing to environmental doping. The carrier mobility value can be extracted by fitting the experimental value of source-to-drain conductance over varying gate voltages [33] . The device presented in Fig. 1d (inset) has a hole-carrier mobility value of 3,342±26 cm 2 Vs −1 and electron carrier mobility of 2,813±11 cm 2 Vs −1 (See Methods and Supplementary Fig. S1 ). Figure 1d also presents a histogram for hole mobility values extracted from 30 different samples. The average hole mobility is 1,771 cm 2 Vs −1 with a standard deviation of 983 cm 2 Vs −1 . These mobility values are several orders of magnitude higher than those of alternative materials such as organic polymer [9] and amorphous materials [10] as expected. More importantly, the unique ambipolar gate response of graphene transistors allows simple implementation of previously mentioned binary modulation schemes as illustrated in Fig. 1e . The amplitude, frequency or phase of the output voltage will be determined by the operating gate bias point of the graphene transistor. For example, amplitude modulation can be achieved by utilizing the transconductance change over the gate voltage difference. Frequency modulation is achieved by interchanging the bias point from a region dominated by electron (or hole) carriers to the charge neutrality point. Similarly, phase modulation is realized by changing the bias point from an electron (or hole) carrier-dominated region to the hole (or electron) carrier-dominated region. Binary and quaternary modulation with a single transistor We next demonstrated the three binary modulation schemes by using the all-graphene circuit. 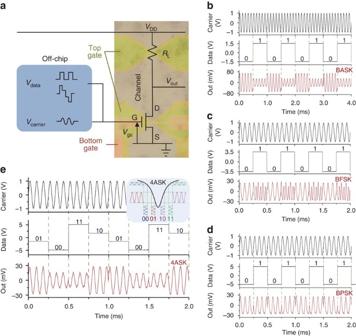Figure 2: Binary and quaternary digital modulations using a single all-graphene transistor. (a) A circuit diagram with a false-colour image of graphene transistors connected in a common-source configuration. TheVdatasignal is the digital data that is encoded onto the carrier signalVcarrier. TheVdatasignal is a square wave for all three binary digital modulation schemes and a four level step-like wave for the 4-ASK modulation scheme. (b) Time domain plot of the BASK.VDDof 1 V is the supply voltage. (c) Time domain plot of the BFSK atVDDof 1 V. (d) Time domain plot of the binary phase-shift keying atVDDof 1 V. (e) A time domain plot of the 4-ASK modulation of carrier signal. The inset is an illustration describing the four operating gate bias points used in 4-ASK.VDDis 1 V. Figure 2a shows the circuit diagram overlaid on a false colour image of the device. Green, grey and red are the respective colours for the top, middle and bottom graphene layers. A graphene transistor was used for the modulation, and another unbiased graphene transistor was used as the load resistor ( R L ) for output ( V out ). The middle graphene layer (grey) serves as the transistor channel, the interconnect between the transistor, the load resistor and the source/drain electrodes. To achieve digital modulation, the carrier wave ( V carrier ), the data bitstream ( V data ) and the DC gate bias ( V gs ) are added together and applied to the top gate (green) of the modulating transistor. Both V gs and V data determine the operating bias point of the transistor and modulate the carrier signal accordingly. The bottom gate (red) delivers additional flexibility to the measurement, and it can also be used to adjust the charge neutrality point ( V Dirac ) if there is environmental doping. Figure 2: Binary and quaternary digital modulations using a single all-graphene transistor. ( a ) A circuit diagram with a false-colour image of graphene transistors connected in a common-source configuration. The V data signal is the digital data that is encoded onto the carrier signal V carrier . The V data signal is a square wave for all three binary digital modulation schemes and a four level step-like wave for the 4-ASK modulation scheme. ( b ) Time domain plot of the BASK. V DD of 1 V is the supply voltage. ( c ) Time domain plot of the BFSK at V DD of 1 V. ( d ) Time domain plot of the binary phase-shift keying at V DD of 1 V. ( e ) A time domain plot of the 4-ASK modulation of carrier signal. The inset is an illustration describing the four operating gate bias points used in 4-ASK. V DD is 1 V. Full size image Figure 2b–d shows plots of three basic binary modulation schemes demonstrated with the all-graphene circuit. For BASK, the sum of V data and V carrier is superimposed on V gs so that the different transconductances on different bias points will allow V carrier to change in amplitude at the output . Binary information of 0 and 1 is successfully represented by the low and high amplitude of carrier signal, respectively ( Fig. 2b ). Similarly, we control V gs and V data to adjust the bias point for both BFSK and BPSK. The values 0 and 1 are successfully differentiated by the doubling in frequencies (BFSK, Fig. 2c ), or by the 180° phase change (BPSK, Fig. 2d ). To the best of our knowledge, this is the first demonstration of BASK using graphene circuit, while previous works have only shown BPSK and BFSK [24] , [28] , [29] . By adding the BASK scheme, the three basic binary schemes have been completed using flexible graphene circuits. We note that the output voltage has a DC component for 0 and 1 because the transistor is operating at different bias points on the gate response curve. The DC component can be filtered out using a high-pass filter and it has been removed for clarity in this paper. Furthermore, by combining BASK and BPSK, a quaternary modulation scheme 4-ASK was demonstrated as shown in Fig. 2e . The inset of Fig. 2e illustrates the four bias points used in the 4-ASK scheme that correspond to 00, 01, 10 and 11. Both the phase and the amplitude information are used to distinguish the quaternary signal that is encoded in the carrier wave. Output of 00, 01, 10 and 11 are represented by low amplitude, 270° phase; high amplitude, 270° phase; high amplitude, 90° phase; and low amplitude, 90° phase in the carrier wave, respectively. A quaternary digital modulation scheme, 4-ASK, uses four points in the constellation diagram ( Fig. 1a ) and doubles the data transfer rate compared with a binary scheme. Importantly, this is the first demonstration of quaternary modulation with just one transistor (excluding the transistor that is used as a resistor), which is not possible in conventional silicon-based modulators. Quadrature phase-shift keying with two graphene transistors A more fundamental quaternary modulation scheme is QPSK, which explores all four quadrants of the constellation. 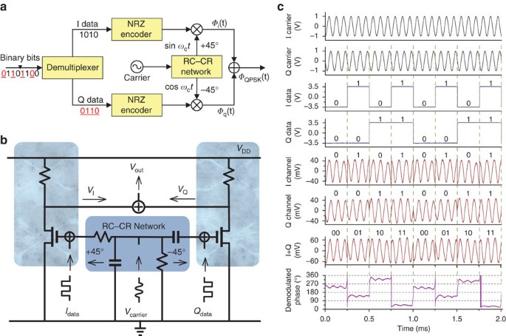Figure 3: QPSK demonstrated with two all-graphene transistors. (a) A conceptual diagram of a conventional QPSK transmitter structure. NRZ encoder is a non-return-to-zero encoder where 1 is represented by a positive voltage state and 0 is represented by a negative voltage state. RC–CR network is the resistance-capacitance–capacitance-resistance phase shift network that generates two orthogonal wave functions with 90° phase difference. (b) An all-graphene circuit diagram of the QPSK system using two transistors. The actual microscopic image of the all-graphene circuit under a blue filter is shown. The transistor dimension is 10 μm×10 μm. (c) Time domain plots of the input and output signals demonstrating QPSK modulation scheme.VDDof 7 V was the supply voltage. Figure 3a shows a typical QPSK transmitter structure used in modern digital communication. A binary data stream is demultiplexed into the in-phase component (I) and the quadrature-phase component (Q). I and Q components are encoded onto two orthogonal basis functions, such as a sine wave and a cosine wave, respectively, before they are summed to generate a QPSK-modulated signal. Figure 3: QPSK demonstrated with two all-graphene transistors. ( a ) A conceptual diagram of a conventional QPSK transmitter structure. NRZ encoder is a non-return-to-zero encoder where 1 is represented by a positive voltage state and 0 is represented by a negative voltage state. RC–CR network is the resistance-capacitance–capacitance-resistance phase shift network that generates two orthogonal wave functions with 90° phase difference. ( b ) An all-graphene circuit diagram of the QPSK system using two transistors. The actual microscopic image of the all-graphene circuit under a blue filter is shown. The transistor dimension is 10 μm×10 μm. ( c ) Time domain plots of the input and output signals demonstrating QPSK modulation scheme. V DD of 7 V was the supply voltage. Full size image Here we used just two transistors with similar gate response in the all-graphene circuit to demonstrate the QPSK modulation ( Fig. 3b ). Actual microscope images under a blue filter are overlaid on top of the circuit diagram. A sinusoidal wave from the function generator was connected to a simple off-chip resistance–capacitance—capacitance–resistance (RC–CR) phase shift network to generate two orthogonal wave functions with 90° phase difference. The sinusoidal input is shifted by +45° in the CR branch and by −45° in the RC branch [34] . Then, each of these signals is summed internally by the function generators with two square waves ( I data and Q data ) and fed to the gates of each transistor (a detailed measurement set-up is shown in the Supplementary Fig. S2 ). The outputs ( V I and V Q ) are then summed to generate the final QPSK-modulated signals. These signal components are plotted in Fig. 3c . The I carrier and the Q carrier are the orthogonal carrier signals. The data bitstream with 00, 01, 10 and 11 is represented by the in-phase component I data and the quadrature-phase component Q data as shown in the plot. Modulating I carrier with I data results in phase changes in I channel and the same applies to Q carrier , Q data and Q channel . Data bit 0 and 1 in I data corresponds to phase of 180° and 0° in I channel . Similarly, Data bit 0 and 1 of Q data corresponds to phase of 90° and 270° in Q channel . The sum of I channel and Q channel is the final output signal ( I + Q ) that has distinct phase shifts of 225°, 135°, 315° and 45°, each corresponding to binary data of 00, 01, 10 and 11. To validate the result, the instantaneous phase information was extracted from the final output signal ( I + Q ) and plotted as demodulated phase ( Fig. 3c , bottom panel). This mathematical form of demodulation was achieved by extracting the phase information from the Hilbert transform of the output signal ( I + Q ). The plot of the demodulated phase indicates a clear distinction of phase shift between different QPSK signals. The carrier to noise ratio (C/N), which is the ratio of signal power to the white-noise power, was found to be 21.1 dB from the frequency spectrum using a conventional signal analysis program (see Methods). The corresponding bit error rate (BER) assuming additive white Gaussian noise channel is much lower than the performance threshold BER of 10 −4 , above which the radio link is considered to be in outage [35] . This confirms the robustness and accuracy of the graphene-based QPSK modulator. From the output signal ( I + Q ) and the input carrier signals, the gain of the QPSK modulator is calculated to be around 0.06, one of largest ever measured with graphene modulators. The gains of our all-graphene binary and quaternary modulators are comparable or larger than all the previous modulator works as shown in the Supplementary Table S1 . Although these gain values are less than 1, in a modern transmitter structure, the amplification of the signal is primarily accomplished by an audio amplifier or a power amplifier, and a gain is not an essential component of the modulator. All-graphene modulator circuits under mechanical strain Last, we examine the performance of all-graphene circuit under mechanical strain ( Fig. 4 ). Frequency modulation (that is, frequency doubling, Supplementary Fig. S3 ) was first evaluated at different bending radii. To quantify the comparison, fast Fourier transform was applied to the doubled output voltage, yielding peaks at ω and 2ω corresponding to the original frequency and the doubled frequency ( Supplementary Fig. S4 ). The ratios of these two peaks, which indicate the spectral purity of the frequency doubling, are plotted as a function of the bending radii in Fig. 4a . Very little change is observed under different bending radii, indicating the robustness in circuit performance under mechanical strain. In addition, various binary and quaternary digital modulation schemes are also successfully demonstrated at maximum strain level of 2.7% (bending radius of 5.5 mm) under the test set-up ( Fig. 4b ). The results further confirm that the transparent all-graphene modulators are fully functional under highly strained conditions. 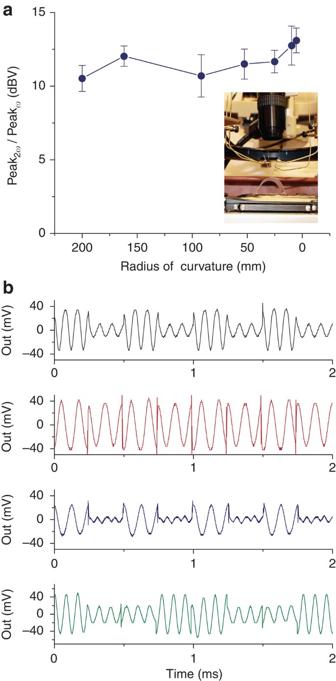Figure 4: Flexible and transparent all-graphene digital modulator circuits under mechanical strain. (a) The plot of the signal amplitude ratio of the original and the doubled frequency as a function of the curvature radius for a graphene frequency doubler. The inset is a photograph of the measurement set-up. (b) Time domain plots of BASK (black), binary phase-shift keying (red), BFSK (blue) and 4-ASK (green) schemes achieved with mechanically strained all-graphene circuits at 5.5 mm radius of curvature (2.7% strain). Figure 4: Flexible and transparent all-graphene digital modulator circuits under mechanical strain. ( a ) The plot of the signal amplitude ratio of the original and the doubled frequency as a function of the curvature radius for a graphene frequency doubler. The inset is a photograph of the measurement set-up. ( b ) Time domain plots of BASK (black), binary phase-shift keying (red), BFSK (blue) and 4-ASK (green) schemes achieved with mechanically strained all-graphene circuits at 5.5 mm radius of curvature (2.7% strain). Full size image The operating principle and technique of flexible and transparent all-graphene modulators described here can be applied to widely used network technologies in today's multimedia and communication devices by either introducing pulse shaping with signal delays or coupling aforementioned modulation schemes [32] . Several recent works also demonstrated voltage gain in graphene transistors showing possibility of graphene-based amplifiers and radiofrequency front-ends in communication system [36] , [37] , [38] . The combination of an efficient modulation method with a reliable radiofrequency front-end will be the key factor in determining the practicality of mobile and flexible apparatus. In conjunction with conventional thin film technology and high-resolution lithography, all-graphene modulator circuits will have a pivotal role in realizing a high speed, mechanically compliant, and transparent electronic system in the near future. Sample fabrication Graphene films used in this work are synthesized using chemical vapour-deposition method on copper foil [39] , [40] , [41] . After the chemical vapour-deposition synthesis, one side of the copper sample with graphene was coated with 950PMMA A2 (Microchem) resist and cured at 180 °C for 1 min. The other side of the sample was exposed to O 2 plasma for 30 s to remove the graphene on that side. The sample was then left in Ammonium persulfate (Sigma Aldrich, 248614-500G) solution (0.025 g ml −1 ) for at least 6 h to completely dissolve away the copper layer. Then the graphene was transferred to a 100-μm thick polyethylene naphthalate substrate. The PMMA coating is removed with acetone and the substrate is rinsed with deionized water several times. The graphene layer was then patterned with a conventional stepper tool (GCA AS200 AutoStepper) using SPR220 3.0 (Microchem) resist. The process temperature was kept under the glass transition temperature of the plastic substrate (120 °C) at all times. After graphene was patterned, 2 nm of Al 2 O 3 was deposited as a buffer layer using e-beam evaporation. Then, 65 nm of Al 2 O 3 was deposited as the dielectric using atomic layer deposition at 80 °C. Another graphene layer was transferred on top of the Al 2 O 3 layer to form the channel layer and then it was patterned with lithography again. E-beam evaporation and atomic layer deposition of Al 2 O 3, with the same thickness as the bottom dielectric, was repeated on top of the channel layer. Final graphene layer was transferred again on top of the dielectric and patterned with lithography to be used as the top gate. Transmittance measurement The transmittance measurement set-up consists of a monochromator (Acton SP2300 triple grating monochromator/spectrograph, Princeton Instruments) coupled with a 250-W tungsten halogen lamp (Hamatsu), a collimator and a photodetector. An iris was used to prevent the photodetector from absorbing the scattered light from the substrate. Optical power measurements were carried out using a 1928-C power meter (Newport) coupled to an ultraviolet-enhanced 918UV Si photodetector (Newport). A blank polyethylene naphthalate substrate was used as a reference for subtraction. DC characterization The contact resistance and the mobility can be extracted by fitting the experimental value of resistance across the source and drain of the graphene transistors with the following equation [33] , where the variables are defined as drain/source voltage V ds , drain/source current I ds , contact resistance R contact , gate capacitance C ox , residual carrier concentration n 0 , the gate voltage V g , the charge neutrality point V Dirac , drain/source width W and length L . Device in Supplementary F S1 indicated a hole mobility of 3,342±26 cm 2 Vs −1 and electron mobility of 2,813±11 cm 2 Vs −1 with residual concentration of n 0 =(2.47±0.01)×1,011 cm −2 and R contact =116.4±0.1 kΩ. For all the cases, the residual concentration matched well with the reported values 2×10 11 cm −2 (ref. 33 ). Notably, the high contact resistance is resulted from series resistance of long graphene strips that have been used as the interconnects between the drain/source electrodes and the contacts. Although the large series resistance currently limits the frequency performance of the devices, this problem can be resolved by partial doping of graphene interconnects in the future. Several works have shown it is possible to lower the graphene sheet resistance significantly by room temperature doping [41] , [42] . Extraction of carrier to noise ratio (C/N) Signal to noise ratio is defined as, This figure characterizes the ratio of the fundamental signal to the noise spectrum. The noise spectrum includes all non-fundamental spectral components such as spurs and the noise floor in the Nyquist frequency range (sampling frequency/2) without the DC component, the fundamental itself and the harmonics. Six harmonics were considered in our calculation. Carrier-to-noise ratio (C/N) (that is, signal-to noise ratio of a -modulated signal) of 21.1 dB was extracted from the fast Fourier transform plot using a conventional program, SBench 6.1 (Spectrum GmbH). The BER from this C/N value is significantly better than the performance threshold of a QPSK system as indicated in the ref. 35 . How to cite this article: Lee, S. et al . Flexible and transparent all-graphene circuits for quaternary digital modulations. Nat. Commun. 3:1018 doi: 10.1038/ncomms2021 (2012).